Synthesis and characterization of tetraphenylammonium salts The phenyl (Ph) group is a representative substituent in the field of organic chemistry as benzene (the parent molecule) is of fundamental importance. Simple Ph-substituted compounds of common chemical elements are well known. However, extensive structural characterization of tetraphenylammonium (Ph 4 N + ) salts has not been reported. Herein, the synthesis of Ph 4 N + salts and their characterization data including the 1 H and 13 C nuclear magnetic resonance (NMR) spectra and the single-crystal X-ray structure have been presented. An intermolecular radical coupling reaction between an aryl radical and a triarylammoniumyl radical cation was conducted to synthesize the target moieties. The Ph 4 N + salts described herein are the simplest tetraarylammonium (Ar 4 N + ) salts known. The results reported herein can potentially help access the otherwise inaccessible non-bridged Ar 4 N + salts, a new class of rigid and sterically hindered organic cations. The elements in groups 13 (B and Al), 14 (C and Si), and 15 (N and P) typically form tetrahedral ions or molecules of the general formula R 4 Z 0 ± 1 , when four identical substituents (R 4 ) are attached to the central element (Z). The charge on the atom Z depends on the group to which it belongs: −1, 0, and +1 for groups 13, 14, and 15, respectively. Compounds of type R 4 Z 0 ± 1 , bearing simple R substituents, are of special importance and considered benchmark compounds. The structural features, physical properties, and chemical reactivities of the other derivatives belonging to this class of compounds were compared with those of the benchmark compounds for a deeper understanding of the compound characteristics. Therefore, for a long time, organic chemists have focused on synthesizing such R 4 Z 0 ± 1 compounds bearing simple R substituents. The compounds of the general formula R 4 Z 0 ± 1 (R = Ph (Ph 4 B − , Ph 4 Al − , Ph 4 C, Ph 4 Si, and Ph 4 P + ; Fig. 1 )) [1] , [2] , [3] , [4] , [5] , [6] are known since long. Ph 4 Si was identified more than 130 years ago. The fundamental properties of these Ph 4 Z 0 ± 1 compounds have been studied extensively over a long period of time. The results serve as references during the study of the corresponding tetraaryl-substituted compounds (Ar 4 Z 0 ± 1 ). Quantum chemical calculations have been conducted for Ph 4 N + [7] . However, the experimental properties of this simple organic cation remain largely unknown. 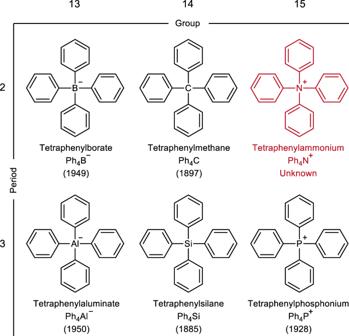Fig. 1: Structures of Ph4-substituted elements belonging to the groups 13–15, Ph4Z0 ± 1. The number in the parentheses indicates the year of synthesis (reported in the literature). Though several researchers have reported the application prospects of the Ph 4 N + salts (Supplementary Table 1 ), the synthetic route followed, and the compound characteristics have not been reported. Fig. 1: Structures of Ph 4 -substituted elements belonging to the groups 13–15, Ph 4 Z 0 ± 1 . The number in the parentheses indicates the year of synthesis (reported in the literature). Full size image It has been reported that the pentatritiated tetraphenylammonium salts ( 1 ; Fig. 2a ) can be formed following the nuclear-chemical method via the tritium β-decay of hexatritiated benzene (C 6 T 6 ) [8] , [9] . The isomorphic co-crystallization data and the radioactivity-based yields have been documented. However, the detailed synthetic procedure and data from experiments conducted for structure identification have not been reported. Bridged Ar 4 N + salts are structurally similar to the Ph 4 N + salts. In 1963, Nesmeyanov synthesized the ( N , N -diphenyl)carbazolium salts ( 2 ; Fig. 2b ) as the first examples of this class of compounds [10] . The key reaction step affording 2 from precursor 3 was the intramolecular N -arylation of triarylamine. The step proceeded via the decomposition of the spatially proximal aryldiazonium moiety. This process resulted in the formation of a 5-membered ring containing a nitrogen atom bearing four aromatic rings. Following the success of the method, a similar cyclization strategy was followed for the synthesis of various ( N , N -diaryl)carbazolium salts [11] , [12] , [13] , [14] , [15] , [16] (such as 4 and 5 ; Fig. 2c ), and sulfide- or amide-bridged Ar 4 N + salts ( 6 [17] and 7 [18] , respectively). Recently, the quaternary ammonium structure of 2 was confirmed using the single-crystal X-ray diffraction technique [13] , [16] . However, none of these bridged Ar 4 N + salts could be converted to Ph 4 N + salts, as there is a dearth of efficient methods that can be used to remove the bridge moieties [17] . Fig. 2: Ar 4 N + salts reported in the literature. Counter anions are depicted in the general form X. a Pentatritiated Ph 4 N + salts ( 1 ) reported without proper structural data. b Synthesis of ( N , N -diphenyl)carbazolium salts ( 2 ) from precursor 3 following the process of intramolecular N -arylation. The bridge moiety indicated in blue must be removed to obtain the Ph 4 N + salts. c Other bridged Ar 4 N + salts such as ( N , N -diphenyl)carbazolium salts ( 4 ) bearing various substituents Y on the aryl groups, spirobicarbazolium salts ( 5 ), sulfide-bridged Ar 4 N + salts ( 6 ), and amide-bridged Ar 4 N + salts ( 7 ) prepared following the intramolecular N -arylation strategy. The bridge moieties are indicated in blue. Full size image Ar 4 N + is a promising organic cation that can be used for developing surfactants, supporting electrolytes, phase-transfer catalysts, and anion-exchange membranes [13] . Also, it is potentially useful for industrial and biological studies. The wide application range of the cation can be attributed to the high chemical stability [14] , [15] and unique rigid structure of the organic cation. Although the bridged Ar 4 N + cations represented by 2 have been studied and characterized, non-bridged Ar 4 N + cations have not been explored because of synthetic limitations. Herein, we report a synthetic strategy for the preparation of Ph 4 N + salts. To the best of our knowledge, this is the first report where the results of structural characteristics of the cation have been reported. Synthetic strategy The direct N -phenylation of triphenylamine ( 8 ; Fig. 3a ) using a Ph cation (or its synthetic equivalent) to form Ph 4 N + is difficult because 8 is weakly nucleophilic (indicated by the low p K aH value (−3.91) [19] recorded during N -protonation). Ph 4 N + salts could not be obtained by reacting 8 with a phenyldiazonium unit [10] . The N -phenylation of 8 using diphenyliodonium [20] or the in-situ-generated benzyne [21] unit was also unsuccessful. We designed the triarylammoniumyl salt ( 9 ; Fig. 3b ) as a novel precursor that could be used for the synthesis of Ph 4 N + to address the problem of low reactivity of 8 . In general, triarylamines can be oxidized to form the corresponding radical cations (referred to as triarylammoniumyls) that exhibit high reactivity. Triphenylammoniumyl easily dimerizes via the para positions of the Ph groups following the process of intermolecular radical coupling to afford tetraphenylbenzidine [22] . The results obtained from quantum chemical calculations revealed that the singly occupied molecular orbital of triphenylammoniumyl was spread over all the Ph rings and the central nitrogen atom [23] . Therefore, we expected that the intermolecular radical coupling reaction involving a triphenylammoniumyl unit and an aryl radical occurs via the nitrogen atom if the Ph group is hindered by steric protection. The tert-butyl and bromo groups were selected as the bulky protecting groups of 9 at the meta- and para-positions, respectively. These groups can exert a large extent of steric hindrance and can be removed at the later stages of the synthetic procedure. Fig. 3: Synthetic strategy followed for the construction of a non-bridged Ar 4 N + structure. 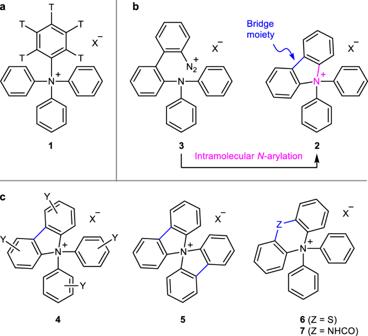Fig. 2: Ar4N+salts reported in the literature. Counter anions are depicted in the general form X.aPentatritiated Ph4N+salts (1) reported without proper structural data.bSynthesis of (N,N-diphenyl)carbazolium salts (2) from precursor3following the process of intramolecularN-arylation. The bridge moiety indicated in blue must be removed to obtain the Ph4N+salts.cOther bridged Ar4N+salts such as (N,N-diphenyl)carbazolium salts (4) bearing various substituents Y on the aryl groups, spirobicarbazolium salts (5), sulfide-bridged Ar4N+salts (6), and amide-bridged Ar4N+salts (7) prepared following the intramolecularN-arylation strategy. The bridge moieties are indicated in blue. a Direct N -phenylation of 8 with a Ph cation is difficult as the N atom is a weak nucleophile. b Intermolecular radical coupling reaction between an aryl radical and the triarylammoniumyl salt 9 bearing bulky protecting groups that exert steric hindrance and block the reactions at the Ph groups. Full size image Synthesis The starting material used for the synthesis of the target was tris[(3,5-di-tert-butyl)phenyl]amine ( 10 ; Fig. 4 ), which was prepared over three steps starting from benzene: Friedel–Crafts reaction, dealkylative bromination, and palladium-catalyzed amination [24] , [25] . The para-brominated compound 11 was formed in 81% yield when 10 was treated with N -bromosuccinimide (NBS). The triarylamine 11 was then activated to form the triarylammoniumyl salt 9 following the one-electron oxidation process using AgBF 4 [26] . It was isolated as a monohydrate in 93% yield. Similar to other triarylammoniumyl salts [22] , 9 was a blue solid. The color could be attributed to the absorption over the visible region (λ max = 797 nm in o -dichlorobenzene). Following this, we investigated the key intermolecular radical coupling reactions. Bis(3,5-di-tert-butyl)benzoyl peroxide ( 13 ) was used as the starting material for the in situ generation of the (3,5-di-tert-butyl)phenyl radical ( 12 ). The formation of the radical proceeded via the process of O–O homolysis, which was followed by the process of decarboxylation [27] . A mixture of 9 and 13 was heated to 120 °C in o -dichlorobenzene in the presence of (2,6-di-tert-butyl)pyridine ( 14 ; used as a base) until the characteristic blue color of 9 disappeared. The reaction conditions were selected from the results of the screening experiments (vide infra). The desired Ar 4 N + salt 15 was successfully formed in a low yield (0.1%), which was then isolated using the normal-phase ion-pair chromatography technique [28] . Under these conditions, 4 g of 9 could be converted to 5 mg of 15 . The byproducts formed during the reaction were triarylamine 11 (11%), solvent adduct 16 (4% based on 13 ), and sterically congested triarylamines 17 (7%) and 18 (8%) possessing ortho-[(3,5-di-tert-butyl)benzoyl]oxy and ortho-(3,5-di-tert-butyl)phenyl groups, respectively. The structures of 17 and 18 were determined using the single-crystal X-ray diffraction technique (Supplementary Tables 2 and 3 , respectively). 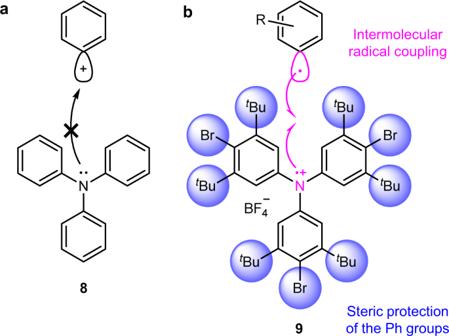Fig. 3: Synthetic strategy followed for the construction of a non-bridged Ar4N+structure. aDirectN-phenylation of8with a Ph cation is difficult as the N atom is a weak nucleophile.bIntermolecular radical coupling reaction between an aryl radical and the triarylammoniumyl salt9bearing bulky protecting groups that exert steric hindrance and block the reactions at the Ph groups. The formation of 17 and 18 indicated that the extent of steric protection provided by the meta-tert-butyl groups in 9 was not sufficient to efficiently inhibit the occurrence of the ortho-substitution reactions at the Ph rings. 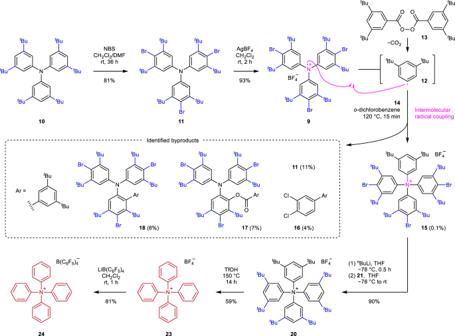Fig. 4: Synthetic scheme for the formation of the Ph4N+salts 23 and 24. Triarylammoniumyl salt9was prepared from10over 2 steps. The intermolecular radical coupling reaction between9and aryl radical12, formed in situ following the thermolysis of the diacyl peroxide13, yielded the Ar4N+salt (15) along with various byproducts (11,16,17, and18). Removal of the bromo and tert-butyl groups in15afforded23, whose counter anion was exchanged to obtain24. Supplementary Table 4 shows the process of reaction condition screening for the intermolecular radical coupling reaction conducted on a small scale using 9 (80–100 mg). When the reaction was conducted in o -dichlorobenzene in the presence of 14 (entry 1), the yield of the desired ammonium salt 15 was 0.12% (determined by 1 H NMR spectroscopic analysis). Although the same yield (0.12%, entry 2) of 15 was obtained when the reaction was carried out in the absence of 14 , it was difficult to purify the product under these conditions as various byproducts were also formed during the process. The use of other solvents in combination with 14 afforded lower (entries 3–10) or undetectable (entries 11–14) yields of 15 , and a complex mixture of compounds which could not be purified or analyzed (entries 16–21). Thus, the reaction conditions presented in entry 1 were used to synthesize 15 from 9 (4 g). We also attempted the intermolecular radical coupling reaction involving 13 and tris[(3,5-di-tert-butyl)phenyl]ammoniumyl BF 4 − ( 19 ; devoid of the p -bromo groups). The latter was prepared following the one-electron oxidation of 10 . However, the desired product tetrakis[(3,5-di-tert-butyl)phenyl]ammonium BF 4 − ( 20 ) could not be isolated as the reaction yielded a complex mixture. Therefore, the removal of all the bromo groups in 15 was carried out following the process of bromine–lithium exchange using n BuLi at −78 °C. The resulting product was protonated with (2,6-di-tert-butyl)pyridinium BF 4 − salt ( 21 ), affording 20 in 90% yield. Since we selected diacyl peroxide 13 as the precursor of aryl radical 12 to introduce the (3,5-di-tert-butyl)phenyl group in 9 , the ammonium nitrogen of 20 was connected to four identical aryl groups. 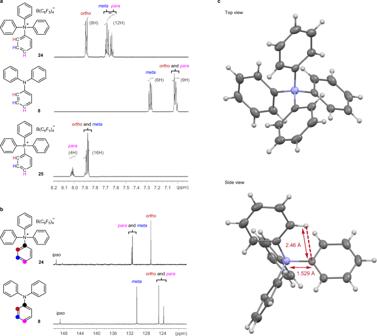Fig. 5: Structural characterization of Ph4N+. aComparison of the1H NMR spectral profiles (600 MHz, (CD3)2CO) recorded for24,8, and25. The number of protons is presented in the parentheses.bComparison of the13C NMR spectral profiles (150 MHz, (CD3)2CO) recorded for24and8.cSingle-crystal X-ray structure of24. All ellipsoids are contoured at the 50% probability level. The counter anion was omitted for clarity. The counter anion of 20 was exchanged to prepare the corresponding B(C 6 F 5 ) 4 − salt ( 22 ), the structure of which was confirmed using the single-crystal X-ray diffraction technique (Supplementary Table 5 ). The final step toward the formation of Ph 4 N + involved the dealkylation of the tert-butyl groups present on the aromatic rings of 20 . All the eight tert-butyl groups could be successfully removed when 20 was heated at 150 °C over a period of 14 h in a solvent amount of trifluoromethanesulfonic acid (TfOH) [29] . The reaction afforded Ph 4 N + BF 4 − ( 23 ) in 59% yield. This result indicates the high stability of Ph 4 N + under extremely harsh acidic conditions. Following the process of counter anion exchange, the BF 4 − salt ( 23 ) was converted to the B(C 6 F 5 ) 4 − salt ( 24 ; yield: 81%; white solid). The purity of the counter anion was confirmed using the 19 F NMR spectroscopy technique. Fig. 4: Synthetic scheme for the formation of the Ph 4 N + salts 23 and 24. Triarylammoniumyl salt 9 was prepared from 10 over 2 steps. The intermolecular radical coupling reaction between 9 and aryl radical 12 , formed in situ following the thermolysis of the diacyl peroxide 13 , yielded the Ar 4 N + salt ( 15 ) along with various byproducts ( 11 , 16 , 17 , and 18 ). Removal of the bromo and tert-butyl groups in 15 afforded 23 , whose counter anion was exchanged to obtain 24 . Full size image 1 H and 13 C NMR spectra The 1 H NMR signals corresponding to 24 (spectra recorded in (CD 3 ) 2 CO) appeared at approximately 7.89, 7.69, and 7.65 ppm. The signal corresponded to the ortho, meta, and para-protons present in the Ph ring, respectively. The 13 C NMR signals corresponding to 24 (spectra recorded in (CD 3 ) 2 CO) appeared at 149.7 (ipso), in the range of 131.4–131.2 (para and meta), and at 126.8 (ortho) ppm. The signals were assigned to the corresponding carbon atoms using the HMQC technique. The 1 H and 13 C NMR signals corresponding to 24 appeared downfield compared to the signals corresponding to 8 (Fig. 5a, b ). The downfield shift can be attributed to the strong inductive effect exerted by the ammonium nitrogen in 24 and the loss of the resonance effect of the lone pair of electrons on nitrogen present in 8 following N- quaternization. The signals corresponding to the meta and para protons present in 24 (at ~7.69 and ~7.65 ppm, respectively) appeared at up-field compared to the signals corresponding to Ph 4 P + B(C 6 F 5 ) 4 − [30] ( 25 ; ~7.88 and ~8.02 ppm for meta and para protons, respectively). The up-field shift may be attributed to the strong anisotropic effects observed in Ph 4 N + . The generation of the strong anisotropic effects can be attributed to the fact that Ph 4 N + is smaller than Ph 4 P + . Similarly, we observed that the signals corresponding to the meta and para protons in Ph 4 C ((CD 3 ) 2 CO; at ~7.29 and ~7.21 ppm, respectively) appeared up-field compared to the signals corresponding to Ph 4 Si (meta and para protons appear at ~7.44 and ~7.48 ppm, respectively; Supplementary Fig. 1 ) [31] . Fig. 5: Structural characterization of Ph 4 N + . a Comparison of the 1 H NMR spectral profiles (600 MHz, (CD 3 ) 2 CO) recorded for 24 , 8 , and 25 . The number of protons is presented in the parentheses. b Comparison of the 13 C NMR spectral profiles (150 MHz, (CD 3 ) 2 CO) recorded for 24 and 8 . c Single-crystal X-ray structure of 24 . All ellipsoids are contoured at the 50% probability level. The counter anion was omitted for clarity. Full size image Single-crystal X-ray structure analysis The single-crystal X-ray diffraction technique was used to analyze the structure of 24 . Analysis of the results proved the quaternary ammonium structure of 24 (Fig. 5c , top view). The counter anion B(C 6 F 5 ) 4 − was omitted for clarity (Supplementary Table 6 ). The Ph 4 N + structure exhibited S 4 -like symmetry and not D 2 d -like symmetry. The result agreed well with the theoretically predicted result [32] . The N–C(sp 2 ) bond length in 24 (present between the Ph 4 N + nitrogen unit and the sp 2 carbon atom) in the Ph group was 1.529 ± 0.003 Å (Fig. 5c , side view). This bond is longer than the N–C(sp 2 ) bonds in (CH 3 ) 3 PhN + , (CH 3 ) 2 Ph 2 N + , (CH 3 )Ph 3 N + , and N , N -diphenylcarbazolium, which were 1.50 [33] , 1.51 [21] , 1.52 [21] , and 1.51–1.52 [16] Å, respectively (data from Cambridge Crystallographic Data Center (CCDC) deposition numbers of 291166, 1433867, 1433868, and 1890475, respectively). The long N–C(sp 2 ) bond in Ph 4 N + indicates the presence of an unusually hindered environment around the ammonium nitrogen atom. The lengths of the bonds formed between the central atom and the sp 2 carbons in Ph 4 C, Ph 4 B − , Ph 4 P + , Ph 4 Si, and Ph 4 Al − were 1.56 [34] , 1.64–1.66 [35] , 1.79 [36] , 1.88 [37] , and 2.00–2.03 [38] Å, respectively. Thus, Ph 4 N + is characterized by the most sterically congested environment among these Ph 4 Z 0 ± 1 , reflecting the difficulty faced during synthesis. The C–N bond length of Ph 4 N + (1.529 Å) was ca. 8% longer than that of 8 (1.419 Å) [39] , whereas the C–P bond length of Ph 4 P + (1.792 Å) was ca. 2% shorter than that of Ph 3 P (1.828 Å) [39] . The shortest distance between the ortho-hydrogen in the Ph unit and the ipso carbon in the adjacent Ph group in Ph 4 N + was 2.46 Å (Fig. 5c , side view). The Van der Waals radii for hydrogen (1.00 Å) and carbon (1.77 Å) indicate that steric repulsion is generated [40] . The corresponding H–C distances in Ph 4 C, Ph 4 B − , and Ph 4 P + were 2.54 [34] , 2.59 [35] , and 2.76 [36] Å, respectively, indicating that the extent of steric repulsion observed in these cases was lower than that observed in Ph 4 N + . The N–C(sp 2 ) bond length in octa-tert-butylated Ph 4 N + salt 22 was in the range of 1.53–1.54 Å and the H–C distance was 2.48 Å. These values are slightly higher than the corresponding values recorded for 24 . This suggested the generation of steric and electronic effects in the presence of the meta-tert-butyl groups in 22 present in the ammonium structure. Initial evaluation of alkaline stability Alkaline stability of Ph 4 N + salt 23 was compared with that of N , N -diphenylcarbazolium PF 6 − salt 2-PF 6 by heating their solutions in CD 3 OD/D 2 O (3:1, containing 5 M KOH) to 80 °C. The 1 H NMR monitoring revealed that 23 was gradually decomposed over 5 days (Supplementary Fig. 2 ) whereas 2-PF 6 almost completely disappeared in 24 h (Supplementary Fig. 4 ). Therefore, 23 exhibited higher alkaline stability than 2-PF 6 . The rapid decrease of the signal assigned to the ortho-protons of 23 suggested that H/D exchange occurred during this experiment [14] . Octa-tert-butylated Ph 4 N + salt 20 exhibited excellent alkaline stability. No apparent spectral change of 20 was observed under the same conditions for 30 days (Supplementary Fig. 5 ). The alkaline stability of 20 can be compared with that of sterically hindered imidazolium salts [41] , which were also inert under similar alkaline conditions. In conclusion, we have synthesized Ph 4 N + salts which are structurally simple non-bridged Ar 4 N + salts. The 1 H and 13 C NMR spectra of the Ph 4 N + salts have been presented. The single-crystal X-ray structure analysis revealed the long N–C bond present in this organic cation. The Ph 4 N + salts described herein are essential benchmarks for non-bridged Ar 4 N + salts. We have confirmed that the non-bridged Ar 4 N + salts we prepared are highly stable under basic conditions. Our findings will encourage further synthetic study of this new class of organic cations which are attractive for diverse applications. The concept of the radical coupling reaction (between a triarylammoniumyl and an aryl radical) reported herein can potentially be applied to the synthesis of various non-bridged Ar 4 N + salts. Further studies need to be conducted to achieve higher product yields. Synthesis of tris[(4-bromo-3,5-di-tert-butyl)phenyl]amine (11) Triarylamine 10 (5.0 g, 8.6 mmol) and NBS (5.0 g, 28 mmol) were added to a mixture of CH 2 Cl 2 /DMF (1:1, 42.0 ml) at room temperature. After 68 h, the reaction mixture was quenched with saturated aqueous Na 2 S 2 O 3 (30 ml) and then extracted with CHCl 3 (200 ml). The organic layer was washed with brine, dried (Na 2 SO 4 ), and filtrated. The filtrate was concentrated under reduced pressure. The crude product was recrystallized from CHCl 3 /MeOH to afford a white solid (5.7 g, 81%). Mp: 246–247 °C; TLC (hexane): RF = 0.50; 1 H NMR (600 MHz, CDCl 3 ): δ 7.11 (s, 6H), 1.48 (s, 54H); 13 C NMR (150 MHz, CDCl 3 ): δ 150.0, 144.9, 121.8, 117.8, 38.4, 31.0; HRMS (ESI-TOF, m / z ): [M] + calcd for C 42 H 60 Br 3 N, 815.2276; found, 815.2278. Synthesis of tris[(4-bromo-3,5-di-tert-butyl)phenyl]ammoniumyl tetrafluoroborate monohydrate (9) A mixture of triarylamine 11 (1.000 g, 1.22 mmol) and AgBF 4 (260 mg, 1.34 mmol) in CH 2 Cl 2 (12.5 ml) was stirred for 2 h at room temperature. The reaction mixture was then filtrated. The filtrate was concentrated under reduced pressure. The residue was washed with hexane to afford a blue solid (1,044 mg, 93%). Mp: 166 °C (decomp. ); UV/vis: λ max 797 nm (in o -dichlorobenzene); HRMS (ESI-TOF, m / z ): [M − BF 4 − H 2 O] + calcd for C 42 H 60 Br 3 N, 815.2276; found, 815.2262; analysis (% calcd, % found for C 42 H 62 BBr 3 F 4 NO): C (54.63, 54.37), H (6.77, 6.48), N (1.52, 1.58). Synthesis of tris[(4-bromo-3,5-di-tert-butyl)phenyl][(3,5-di-tert-butyl)phenyl]ammonium tetrafluoroborate (15) A mixture of triarylammoniumyl salt 9 (1.000 g, 1.08 mmol), diacyl peroxide 13 (1.550 g, 3.321 mmol), and pyridine 14 (250 μl, 1.11 mmol) in o -dichlorobenzene (8.5 ml) was heated to 120 °C for 15 min. Then, the reaction mixture was cooled to room temperature and filtered (CHCl 3, 20 ml). This reaction procedure was repeated another three times to obtain a set of four filtrate solutions. The combined filtrate solution was passed through NaBF 4 -treated silica gel to afford Fraction A (CHCl 3 as an eluent, 350 ml) followed by Fraction B (CHCl 3 /MeOH = 90:10 as an eluent, 400 ml). Concentration of Fractions A and B under reduced pressure afforded Residues A and B, respectively. Residue B was purified by ion-pair column chromatography (NaBF 4 -treated silica gel, CHCl 3 /MeOH = 95:5) followed by preparative thin layer ion-pair chromatography [NaBF 4 -treated silica gel TLC plate, 0.50 mm thick, three times (CHCl 3 /MeOH = 90:10, hexane/EtOAc = 30:70, and hexane/EtOAc = 40:60 for the first, the second, and the third chromatography, respectively)] to afford 15 as an off-white solid (4.97 mg, 0.11%). TLC (NaBF 4 -treated silica gel, CHCl 3 /MeOH = 90:10): RF = 0.40; 1 H NMR (600 MHz, CDCl 3 ): δ 7.60 (t, J = 1.5 Hz, 1H), 7.47 (s, 6H), 7.23 (d, J = 1.5 Hz, 2H), 1.48 (s, 54H), 1.28 (s, 18H); 1 H NMR (600 MHz, CD 3 OD): δ 7.78 (t, J = 1.4 Hz, 1H), 7.47 (s, 6H), 7.28 (d, J = 1.4 Hz, 2H), 1.48 (s, 54H), 1.28 (s, 18H); 13 C NMR (150 MHz, CDCl 3 ): δ 154.6, 152.9, 147.9, 146.3, 127.5, 124.8, 122.7, 119.3, 39.3, 35.9, 31.3, 30.6; 19 F NMR (376 MHz, CDCl 3 ): δ −154.4; HRMS (ESI-TOF, m / z ): [M − BF 4 ] + calcd for C 56 H 81 Br 3 N, 1004.3919; found, 1004.3898. Partial purification of Residue A by column chromatography (silica gel, hexane/CHCl 3 = 100:0 to 90:10 to 80:20) afforded Fraction A1 (containing compounds 11 , 16 , and 18 ) and Fraction A2 (containing compound 17 ). Further purification of Fraction A1 using recycling preparative HPLC afforded 11 (404 mg, 11%), 16 (348 mg, 3.9% based on 13 ), and 18 (366 mg, 8.4%). Further purification of Fraction A2 (silica gel, hexane/CHCl 3 = 90:10) followed by recrystallization (hexane/CHCl 3 ) afforded 17 (312 mg, 6.9%). Synthesis of tris[(3,5-di-tert-butyl)phenyl]ammoniumyl tetrafluoroborate dihydrate (19) A mixture of triarylamine 10 (150 mg, 0.26 mmol) and AgBF 4 (60 mg, 0.31 mmol) in CH 2 Cl 2 (2.5 ml) was stirred for 1.5 h at room temperature. The reaction mixture was then filtrated. The filtrate was concentrated under reduced pressure. The residue was washed with hexane to afford a blue solid (155 mg, 85%). Mp: 170 °C (decomp. ); UV/vis: λ max 353 nm (in o -dichlorobenzene); HRMS (ESI-TOF, m / z ): [M − BF 4 − 2H 2 O] + calcd for C 42 H 63 N, 581.4961; found, 581.4973; analysis (% calcd, % found for C 42 H 67 BF 4 NO 2 ): C (71.57, 71.14), H (9.58, 9.18), N (1.99, 1.91). Synthesis of tetrakis[(3,5-di-tert-butyl)phenyl]ammonium tetrafluoroborate (20) n BuLi solution in hexane (1.56 M, 110 μl, 172 μmol) was added to a solution of Ar 4 N + salt 15 (5.8 mg, 5.3 μmol) in THF (1.7 ml) at −78 °C. After 25 min, the reaction mixture was quenched by adding 21 (47.0 mg, 168 μmol) under N 2 flow. After 5 min, the reaction mixture was allowed to warm to room temperature and concentrated under reduced pressure. The residue was suspended in CH 2 Cl 2 (10 ml). The resulting suspension was filtered, and the filtrate was concentrated under reduced pressure. The residue was purified by ion-pair column chromatography (NaBF 4 -treated silica gel, CHCl 3 /MeOH = 100:0 to 90:10) followed by preparative thin layer ion-pair chromatography (NaBF 4 -treated silica gel TLC plate, 0.50 mm thick, CHCl 3 /MeOH = 90:10) to afford an off-white solid (4.1 mg, 90%). TLC (NaBF 4 -treated silica gel, CHCl 3 /MeOH = 90:10): RF = 0.35; 1 H NMR (600 MHz, CDCl 3 ): δ 7.53–7.51 (m, 4H), 7.33–7.30 (m, 8H), 1.25 (s, 72H); 1 H NMR (600 MHz, CD 3 OD): δ 7.67 (t, J = 1.6 Hz, 4H), 7.42 (d, J = 1.6 Hz, 8H), 1.26 (s, 72H); 13 C NMR (100 MHz, CDCl 3 ): δ 153.9, 148.5, 124.2, 119.7, 35.7, 31.3; 19 F NMR (565 MHz, CDCl 3 ): δ −154.6; HRMS (ESI-TOF, m / z ): [M − BF 4 ] + calcd for C 56 H 84 N, 770.6604; found, 770.6587. Synthesis of tetrakis[(3,5-di-tert-butyl)phenyl]ammonium tetrakis(pentafluorophenyl)borate (22) A solution of Ar 4 N + salt 20 (1.47 mg, 1.7 μmol) and LiB(C 6 F 5 ) 4 –Et 2 O (4.2 mg, 5.6 μmol as a 1:1 complex) in CH 2 Cl 2 (500 μl) was stirred for 25 min at room temperature. The reaction mixture was directly purified by column chromatography (diol-functionalized silica gel, CH 2 Cl 2 ) to afford an off-white solid (2.19 mg, 88%). TLC (CHCl 3 /acetone = 80:20): RF = 0.17; 1 H NMR (600 MHz, CDCl 3 ): δ 7.52 (t, J = 1.4 Hz, 4H), 7.29 (d, J = 1.4 Hz, 8H), 1.22 (s, 72H); 13 C NMR (150 MHz, CDCl 3 ): δ 153.9, 148.4, 124.2, 119.8, 35.6, 31.2; 19 F NMR (565 MHz, CDCl 3 ): δ −132.5, −163.5, −167.0; HRMS (ESI-TOF, m / z ): [M − B(C 6 F 5 ) 4 ] + calcd for C 56 H 84 N, 770.6604; found, 770.6589. Suitable crystals for X-ray analysis were obtained by recrystallization (acetone/MeOH). Synthesis of tetraphenylammonium tetrafluoroborate (23) A solution of Ar 4 N + salt 20 (3.92 mg, 4.6 μmol) in TfOH (2.0 ml) was heated to 150 °C for 14 h, and then cooled to room temperature. The reaction mixture was concentrated under reduced pressure, and the residue was dissolved in H 2 O (6 ml). The solution was neutralized with aqueous NaOH (0.5 M), saturated with NaBF 4 (~3 g), and extracted with CHCl 3 (10 × 5 ml). The organic layer was dried (Na 2 SO 4 ) and filtrated. The filtrate was concentrated under reduced pressure. Preparative thin layer ion-pair chromatography (NaBF 4 -treated silica gel TLC plate, 0.5 mm thick, CHCl 3 /MeOH = 90:10) afforded an off-white solid (1.10 mg, 59%). TLC (NaBF 4 -treated silica gel, CHCl 3 /MeOH = 95:5): RF = 0.45; 1 H NMR (600 MHz, CD 3 OD): δ 7.76–7.70 (m, 8H), 7.65–7.55 (m, 12H); 13 C NMR (150 MHz, CD 3 OD): δ 150.0, 131.6, 131.4, 127.0; 19 F NMR (565 MHz, CDCl 3 ): δ −153.8; IR: 2958, 2920, 2851, 1733, 1477, 1452, 1259, 1091, 1043, 1022, 996, 799, 757, 692, 631, 491, 431, 412 cm −1 ; HRMS (ESI-TOF, m / z ): [M − BF 4 ] + calcd for C 24 H 20 N, 322.1596; found, 322.1602. Synthesis of tetraphenylammonium tetrakis(pentafluorophenyl)borate (24) A solution of Ar 4 N + salt 23 (1.10 mg, 2.7 μmol) and LiB(C 6 F 5 ) 4 –Et 2 O (4.1 mg, 5.4 μmol as a 1:1 complex) in CH 2 Cl 2 (500 μl) was stirred for 1 h at room temperature. The reaction mixture was directly purified by column chromatography (diol-functionalized silica gel, CH 2 Cl 2 ) to afford a white solid (2.17 mg, 81%). TLC (diol-functionalized silica gel, CHCl 3 ): RF = 0.31; 1 H NMR [600 MHz, (CD 3 ) 2 CO]: δ 7.91–7.87 (m, 8H), 7.72–7.67 (m, 8H), 7.67–7.62 (m, 4H); 13 C NMR [150 MHz, (CD 3 ) 2 CO]: δ 149.7, 131.4, 131.2, 126.8; 19 F NMR (565 MHz, CDCl 3 ): δ −132.4, −163.1, −166.8; IR: 2955, 2917, 2850, 1712, 1643, 1513, 1462, 1275, 1086, 979, 775, 756, 746, 692, 661, 418 cm −1 ; HRMS (ESI-TOF, m / z ): [M − B(C 6 F 5 ) 4 ] + calcd for C 24 H 20 N, 332.1596; found, 332.1606. Suitable crystals for X-ray analysis were obtained by recrystallization (acetone/MeOH).